Grail controls Th2 cell development by targeting STAT6 for degradation T helper (Th)-2 cells are the major players in allergic asthma; however, the mechanisms that control Th2-mediated inflammation are poorly understood. Here we find that enhanced expression of Grail , an E3 ubiquitin ligase, in Th2 cells depends on interleukin (IL)-4-signalling components, signal transducer and activator of transcription 6 (Stat6) and Gata3, that bind to and transactivate the Grail promoter. Grail deficiency in T cells leads to increased expression of Th2 effector cytokines in vitro and in vivo and Grail-deficient mice are more susceptible to allergic asthma. Mechanistically, the enhanced effector function of Grail-deficient Th2 cells is mediated by increased expression of Stat6 and IL-4 receptor α-chain. Grail interacts with Stat6 and targets it for ubiquitination and degradation. Thus, our results indicate that Grail plays a critical role in controlling Th2 development through a negative feedback loop. CD4 + T helper (Th) cells are critical components in adaptive immunity. After activation, CD4 + Th cells differentiate into various effector subsets characterized by expression of lineage-specific transcriptional factors and cytokines that determine their effector functions [1] . Th2 cells produce interleukin (IL)-4, IL-5 and IL-13, which are important for immunity against extracellular parasites and provide help to B cells for antibody production [1] , [2] . However, abnormal Th2 activation is responsible for allergic inflammatory diseases such as asthma [3] . Work in the past decade has revealed complex regulation of the Th2 cell differentiation programme [4] , [5] , [6] . The cytokine IL-4 is the determining factor for Th2 differentiation [4] , [6] , [7] . IL-4 binding to the IL-4 receptor (IL-4R) results in signal transducer and activator of transcription 6 (Stat6) recruitment, phosphorylation, dimerization and translocation to the nucleus, where Stat6 activates the transcription factor Gata3, which is considered as a Th2 master regulator [8] , [9] , [10] . T-cell receptor (TCR) and costimulatory receptor signals are important for early IL-4 production during Th2 differentiation by regulating expression of the nuclear factor of activated T cells (NFATs), activating protein-1 protein JunB and interferon regulatory factor 4 (IRF4) [11] , [12] , [13] , [14] , [15] , [16] . In addition to IL-4, IL-2 and IL-21 cytokines are also involved in the initiation of Th2 differentiation [17] , [18] . However, the factors and mechanisms that control abnormal Th2 development and protect from Th2-mediated autoimmunity are poorly understood. Recent evidence has suggested that E3 ubiquitin ligases, including Cbl-b, Itch and Grail, are crucial regulators of T-cell activation [19] . Grail is a type I transmembrane protein localized to the endosomal compartment whose expression is associated with T-cell anergy induction [20] . Recently, we reported that Grail knockout (KO) mice were resistant to immune tolerance induction in vitro and in vivo [21] . In addition to tolerant T cells, Grail mRNA is upregulated during normal T-cell activation, suggesting that Grail function might not be restricted to T-cell anergy [21] , [22] . Grail expression has also been linked to hyporesponsive Th2 cells in a model of chronic murine schistosomiasis [23] . In fact, overexpression of Grail in T-cell hybridomas dramatically limits production of Th2 essential cytokines such as IL-2 and IL-4 (ref. 20 ), suggesting the role of Grail in controlling Th2 programming. In the current study, high expression of Grail in in vitro differentiated Th2 cells compared with other Th lineages is selectively induced upon IL-4 stimulation in a time-dependent manner and depends on Th2-specific factors Stat6 and Gata3 that bind to and transactivate the Grail promoter. Grail deficiency in T cells leads to enhanced Th2 development in vitro and in vivo ; Grail KO mice are more susceptible to allergic asthma. Both naïve T cells and Th2-polarized cells from Grail KO mice exhibit increased Stat6 transcription factor expression. Moreover, Grail interacts with Stat6 and promotes Stat6 ubiquitination and degradation. Our results suggest an important link between the Th2-specific expression of Grail and its role in control of Th2 development and Th2-mediated pathogenesis and immunity. Regulation of Grail expression in Th2 cells Although it is known that Grail is expressed in anergic cells generated both in vivo and in vitro , its expression is also upregulated during T-cell activation [21] , [22] . To further dissect the role of Grail in Th cell activation and differentiation, fluorescence-activated cell-sorted (FACS) naïve CD4 + CD25 − CD62L hi CD44 lo T cells were differentiated in vitro under Th0, Th1, Th2 and Th17 polarizing conditions and analysed for Grail mRNA expression. Consistent with a previous study, which showed upregulation of Grail in Th2 cells during chronic schistosomiasis [23] , Grail mRNA level was significantly increased in Th2 cells compared with other T-helper subsets ( Fig. 1a ), suggesting a possible role of Grail in Th2 cell development. 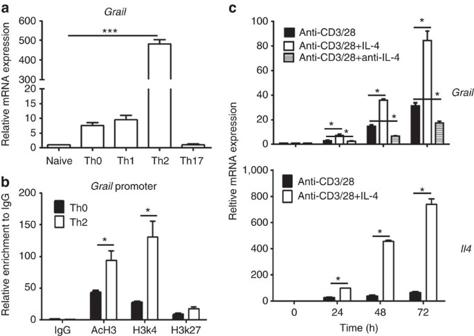Figure 1: Selective expression ofGrailin T helper 2 cells. (a) Naïve CD4+CD25−CD62LhiCD44loT cells from C57BL/6 mice were activated with anti-CD3 and anti-CD28 and cultured for 4 days under Th0, Th1, Th2 and Th17 polarizing cell conditions.GrailmRNA expression was analysed by qRT–PCR analysis. (b) Chromatin immunoprecipitation analysis of histone H3 acetylation (AcH3), trimethyl histone H3 lysine 4 (H3k4) and trimethyl histone H3 lysine 27 (H3K27) methylation atGrailpromoter locus in CD4+T cells polarized under Th0 and Th2 conditions. The data from each replicate were normalized to the input control and the graphs represent fold enrichment of the indicated proteins to control antibody (rabbit IgG) at the designated locus. (c) Naïve CD4+T cells were cultured under indicated conditions andGrailandIl4mRNA expression levels were analysed in different time points by qRT–PCR. The data shown inaandcwere normalized by the expression of a reference geneActb. The results shown are mean±s.e.m. *P<0.05, ***P<0.001, Student’st-test was performed to detect between-group differences.t-test. The data are representative of at least three independent experiments with consistent results. Figure 1: Selective expression of Grail in T helper 2 cells. ( a ) Naïve CD4 + CD25 − CD62L hi CD44 lo T cells from C57BL/6 mice were activated with anti-CD3 and anti-CD28 and cultured for 4 days under Th0, Th1, Th2 and Th17 polarizing cell conditions. Grail mRNA expression was analysed by qRT–PCR analysis. ( b ) Chromatin immunoprecipitation analysis of histone H3 acetylation (AcH3), trimethyl histone H3 lysine 4 (H3k4) and trimethyl histone H3 lysine 27 (H3K27) methylation at Grail promoter locus in CD4 + T cells polarized under Th0 and Th2 conditions. The data from each replicate were normalized to the input control and the graphs represent fold enrichment of the indicated proteins to control antibody (rabbit IgG) at the designated locus. ( c ) Naïve CD4 + T cells were cultured under indicated conditions and Grail and Il4 mRNA expression levels were analysed in different time points by qRT–PCR. The data shown in a and c were normalized by the expression of a reference gene Actb . The results shown are mean±s.e.m. * P <0.05, *** P <0.001, Student’s t -test was performed to detect between-group differences. t -test. The data are representative of at least three independent experiments with consistent results. Full size image We next checked whether this increase is mediated by active transcriptional machinery in the Grail promoter region. Acetyl histoneH3 lysine9/14(AcH3) and histone H3 lysine 4 methylation (H3k4) are typically associated with active transcription, whereas H3 lysine 27 methylation (H3k27) is mainly associated with gene silencing [24] , [25] . Naïve CD4 + T cells differentiated under Th0 and Th2 conditions in vitro were assessed for abundance of AcH3, H3k4 and H3k27 in Grail promoter by chromatin immunoprecipitation (ChIP) assay. The Grail promoter region was significantly enriched with active histone modifications (AcH3 and H3k4) in the Th2 cells compared with Th0 cells ( Fig. 1b ), suggesting a role for IL-4 signalling in regulation of chromatin modification in the Grail locus. The Il4 gene promoter region was analysed as positive control ( Supplementary Fig. 1 ). To further dissect the role of IL-4 in Grail regulation, we analysed Grail expression in naïve CD4 + T cells activated with anti-CD3/28 and treated with IL-4 or anti-IL-4 for 24, 48 or 72 h. This analysis showed that Grail was expressed as early as 24 h after T-cell activation and IL-4 was essential for this induction, because blockade of IL-4 in Th0 condition decreased Grail expression ( Fig. 1c ). Grail expression was further increased in a time-dependent manner and correlated with the level of Il4 expression. The above results suggest that Grail is highly expressed in Th2 cells in an IL-4-dependent manner. As Grail expression is significantly increased upon IL-4 treatment, we assessed whether its expression is regulated by Stat6, a transcription factor that promotes Th2 differentiation in an IL-4-dependent manner [26] . Naïve CD4 + T cells from wild-type (WT) and Stat6 KO mice were cultured under Th2 conditions for 4 days and then assessed for Grail mRNA expression ( Fig. 2a ). Absence of Stat6 led to a significantly decreased expression of Grail in Th2 cells. Similarly, we found significantly low mRNA level of Grail in Stat6-deficient memory CD4 + T cells compared with WT cells ( Supplementary Fig. 2a ). To determine the exact role of Stat6 in regulating Grail expression, we assessed the status of histone modifications at the Grail promoter locus in WT and Stat6-deficient Th2 cells by ChIP analysis. As expected, Stat6-deficient Th2 cells showed decreased active histone modifications (AcH3 and H3k4) and increased abundance of inactive H3k27 modifications in the Grail promoter locus ( Fig. 2b ). To check if this effect is mediated by direct binding of Stat6 to the Grail promoter locus, we performed ChIP assay with Stat6 and control antibodies ( Fig. 2c ). Stat6 binding was enriched in the Th2 cells compared with Th0 cells in the Grail promoter. Apart from Stat6, we also checked binding of Gata3, a transcription factor downstream of Stat6 and also IRF4 and Jun B transcription factors, which are known to have important functions in Th2 cell differentiation [14] , [16] ( Fig. 2c ). Similar to Stat6, Gata3 showed increased binding to the Grail promoter in Th2 cells compared with Th0 cells, whereas we observed moderate binding of IRF4 and JunB to Grail promoter locus, which was not Th2 cell specific ( Fig. 2c ). Binding of the above factors was also analysed at various control loci ( Supplementary Fig. 2b ). The above factors were then overexpressed by retroviral transduction into naïve CD4 + T lymphocytes. Upon overexpression, both Stat6 and Gata3 facilitated a significant increase in Grail expression, whereas IRF4 and JunB did not ( Fig. 2d , upper panel). Expression of Il4 was also checked to validate our overexpression system ( Fig. 2d , lower panel). 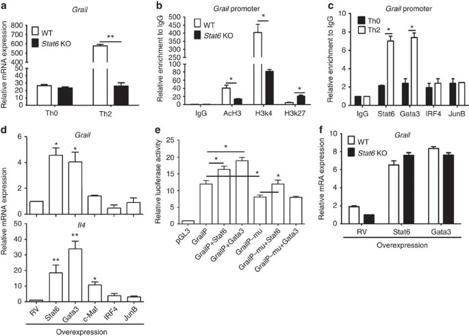Figure 2: Regulation ofGrailexpression in Th2 cells. (a) Naïve CD4+T cells from WT andStat6KO mice were cultured for 4 days under Th0 and Th2 conditions and analysed forGrailmRNA expression by qRT–PCR. (b) ChIP analysis of histone H3 acetylation (AcH3), trimethyl histone H3 lysine 4 (H3k4) and trimethyl histone H3 lysine 27 (H3k27) atGrailpromoter locus in CD4+T cells from WT andStat6KO mice polarized under Th2 condition. The data from each replicate were normalized to the input control and the graphs represent fold enrichment of the indicated proteins to control antibody (rabbit IgG) at the designated locus. (c) ChIP assay to check binding of indicated transcription factors to theGrailpromoter locus in naïve CD4+T cells polarized under Th0 and Th2 conditions. (d)GrailandIl4mRNA expression in naïve CD4+T lymphocytes infected with bicistronic retroviruses expressing the indicated factors. (e) Luciferase assay in EL-4 cells transfected withGrailpromoter (Grail-P) containing luciferase vector or with a mutated Gata3 site (GrailP-mu) promoter along with vectors containing the indicated factors. Luciferase activity is expressed relative to the expression of co-transfected renilla luciferase plasmid as a control for transfection efficiency. Relative luciferase units are expressed as a fold difference to the control (vector only, pGL3) value. (f)GrailmRNA expression in naïve CD4+T lymphocytes from WT andStat6KO mice infected with bicistronic retroviruses expressing the indicated factors. The data shown ina,dandfwere normalized by the expression of a reference geneActb. The results shown are mean±s.e.m. *P<0.05, **P<0.01, Student’st-test was performed to detect between-group differences. The data are representative of least three independent experiments with consistent results. Figure 2: Regulation of Grail expression in Th2 cells. ( a ) Naïve CD4 + T cells from WT and Stat6 KO mice were cultured for 4 days under Th0 and Th2 conditions and analysed for Grail mRNA expression by qRT–PCR. ( b ) ChIP analysis of histone H3 acetylation (AcH3), trimethyl histone H3 lysine 4 (H3k4) and trimethyl histone H3 lysine 27 (H3k27) at Grail promoter locus in CD4 + T cells from WT and Stat6 KO mice polarized under Th2 condition. The data from each replicate were normalized to the input control and the graphs represent fold enrichment of the indicated proteins to control antibody (rabbit IgG) at the designated locus. ( c ) ChIP assay to check binding of indicated transcription factors to the Grail promoter locus in naïve CD4 + T cells polarized under Th0 and Th2 conditions. ( d ) Grail and Il4 mRNA expression in naïve CD4 + T lymphocytes infected with bicistronic retroviruses expressing the indicated factors. ( e ) Luciferase assay in EL-4 cells transfected with Grail promoter (Grail-P) containing luciferase vector or with a mutated Gata3 site (GrailP-mu) promoter along with vectors containing the indicated factors. Luciferase activity is expressed relative to the expression of co-transfected renilla luciferase plasmid as a control for transfection efficiency. Relative luciferase units are expressed as a fold difference to the control (vector only, pGL3) value. ( f ) Grail mRNA expression in naïve CD4 + T lymphocytes from WT and Stat6 KO mice infected with bicistronic retroviruses expressing the indicated factors. The data shown in a , d and f were normalized by the expression of a reference gene Actb . The results shown are mean±s.e.m. * P <0.05, ** P <0.01, Student’s t -test was performed to detect between-group differences. The data are representative of least three independent experiments with consistent results. Full size image To further determine whether the binding of Stat6 and Gata3 to the Grail promoter resulted in its transactivation, we performed dual luciferase reporter assay by overexpression of the above factors along with the Grail promoter construct in EL-4 cells. As expected, both Stat6 and Gata3 transactivated the Grail promoter ( Fig. 2e ). To further assess whether Gata3 is required for Stat6 activity, we used Grail promoter with a mutated Gata3-binding site (GrailP-mu; Fig. 2e ). We found that endogenous activity of Grail promoter was significantly lower when Gata3 site was mutated, suggesting that Gata3 is required for Grail expression. However, Stat6 is still able to transactivate the GrailP-mu. Overall, these data suggest that Stat6 and Gata3 could independently regulate Grail expression. To further confirm these observations, we overexpressed Stat6 and Gata3 in both WT and Stat6-deficient cells. We found that overexpression of either of these two factors can rescue Grail expression in Stat6-deficient cells ( Fig. 2f ). We also checked the expression of Il4 , Stat6 and Gata3 to validate our overexpression system ( Supplementary Fig. 2c ). Together, these findings indicate that Grail expression is induced by IL-4 and both Stat6 and Gata3 are sufficient to induce Grail . Enhanced Th2 response by Grail-deficient T cells in vitro The enhanced Grail expression in Th2 cells led us to further check the role of Grail in Th2 cell development. Naive CD4 + T cells from WT and Grail KO mice were activated with anti-CD3 and anti-CD28 in the presence or absence of IL-4 ( Fig. 3a ). Enhanced expression level of the Th2-specific factors was detected in both IL-4-treated and untreated Grail-deficient cells compared with WT cells. Similarly, in vitro differentiated Grail-deficient Th0 and Th2 cells showed increased expression of Th2-specific factors (IL-4, IL-5, IL-13 and Gata3 ) compared with WT cells ( Fig. 3b,c ). As expected, Grail-deficient Th2 cells showed increased active histone modifications (AcH3 and H3k4) in the Il4 and Gata3 promoter locus and decreased abundance of inactive H3k27 modifications ( Supplementary Fig. 3 , right panel), suggesting that Grail-deficient cells more profoundly acquire a Th2 phenotype. 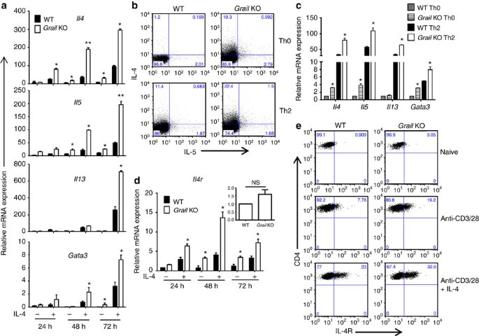Figure 3: Grail deficiency upregulates Th2 cytokines and IL-4 receptorin vitro. (a) Naïve CD4+T cells from WT andGrailKO mice were activated with anti-CD3 and anti-CD28 in the presence or absence of IL-4 for 24, 48 and 72 h and analysed for expression of Th2-specific genes by qRT–PCR. (b,c) Naïve CD4+T cells from WT andGrailKO mice were cultured under Th2 conditions for 4 days and analysed for IL-4 and IL-5 expression by intracellular cytokine staining (b). Numbers in dot plot quadrants represent the percentages. mRNA levels of the indicated genes were analysed (c). (d) Naïve CD4+T cells from WT andGrailKO mice were activated as inaand analysed forIl4rexpression by qRT–PCR. (e) Naïve CD4+T cells from WT andGrailKO mice were activated for 48 h as indicated and analysed for IL-4R expression by FACS. Numbers in dot plot quadrants represent the percentages. The data shown ina,canddwere normalized by the expression of a reference geneActb. The results shown are mean±s.e.m. *P<0.05, **P<0.01, Student’st-test was performed to detect between-group differences. The data are representative of at least three independent experiments with consistent results. Figure 3: Grail deficiency upregulates Th2 cytokines and IL-4 receptor in vitro. ( a ) Naïve CD4 + T cells from WT and Grail KO mice were activated with anti-CD3 and anti-CD28 in the presence or absence of IL-4 for 24, 48 and 72 h and analysed for expression of Th2-specific genes by qRT–PCR. ( b , c ) Naïve CD4 + T cells from WT and Grail KO mice were cultured under Th2 conditions for 4 days and analysed for IL-4 and IL-5 expression by intracellular cytokine staining ( b ). Numbers in dot plot quadrants represent the percentages. mRNA levels of the indicated genes were analysed ( c ). ( d ) Naïve CD4 + T cells from WT and Grail KO mice were activated as in a and analysed for Il4r expression by qRT–PCR. ( e ) Naïve CD4 + T cells from WT and Grail KO mice were activated for 48 h as indicated and analysed for IL-4R expression by FACS. Numbers in dot plot quadrants represent the percentages. The data shown in a , c and d were normalized by the expression of a reference gene Actb . The results shown are mean±s.e.m. * P <0.05, ** P <0.01, Student’s t -test was performed to detect between-group differences. The data are representative of at least three independent experiments with consistent results. Full size image Furthermore, elevated expression of Th2 cytokines by Grail-deficient Th0 and Th2 cells functionally associated with enhanced IL-4R expression ( Fig. 3d,e and Supplementary Fig. 4a ), because IL-4 blockade under Th0 condition diminished difference in Il4r expression between WT and Grail-deficient cells. Interestingly, Grail deficiency in naïve T cells already led to a slight enhancement in IL-4R expression, which was significantly enhanced 24 h after activation and peaked at 48 h ( Fig. 3d,e ). In addition, analysis of Il4r promoter locus in naïve Grail-deficient CD4 + T cells showed both active and inactive histone modifications ( Supplementary Fig. 3 ), suggesting that in the absence of Grail, IL-4R is poised for rapid transcription. Upon Th2 differentiation Il4r promoter locus still maintained a more open chromatin configuration in Grail-deficient cells compared with WT ( Supplementary Fig. 3 ). IL-2- and IL-21-dependent Th2 responses in Grail KO T cells The above results indicate the role of Grail in regulation of IL-4R expression at early stage of Th2 cell programming. In addition, we found enhanced expression of Nfatc1 in Grail-deficient T cells in an IL-4-dependent manner ( Supplementary Fig. 4b ). Role of NFATc1 is well known in regulation of the cytokines IL-2 and IL-21, which play a role in early Th2 development [17] , [18] . As expected, mRNA expression of both Il2 and Il21 was increased in Grail-deficient CD4 + T cells as early as 24 h of activation with anti-CD3/28 in an IL-4-dependent manner, because IL-4 blockade diminished this difference ( Fig. 4a and Supplementary Fig. 4b ). To check whether the increased IL-2 and IL-21 levels aid in the increased Th2 responses seen in Grail KO Th2 cells, we blocked both IL-2 and IL-21 expression in WT and Grail KO CD4 + T cells by respective antibodies for 48 h. We found that blockade of either IL-2 or IL-21 led to decreased expression of Th2 cytokines Il4 , Il5 , Il13 and Il4r more prominently in Grail KO cells compared with WT cells ( Fig. 4b ). As Grail resides in the endosome, we next treated the WT or Grail-deficient T cells activated in the presence or absence of IL-4 with an endosome inhibitor Latrunculin B. mRNA analysis 48 h post treatment showed that expression of Il4r and most Th2-specific genes were upregulated upon Latrunculin B treatment ( Fig. 4c,d ), supporting the critical role of Grail in controlling Th2 development. 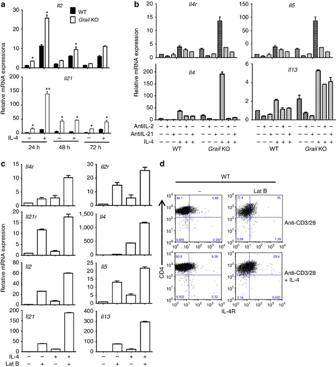Figure 4: Grail controls IL-4 receptor expression in Th2 cells. (a) Naïve CD4+T cells from WT andGrailKO mice were activated with anti-CD3 and anti-CD28 in the presence or absence of IL-4 for 24, 48 and 72 h and analysed for expression ofIl2andIl21by qRT–PCR. (b) Naïve CD4+T cells from WT andGrailKO mice were activated with anti-CD3 and anti-CD28 along with the indicated conditions for 48 h and the mRNA expression of the indicated genes was analysed. (c,d) Naïve CD4+T cells from WT mice were activated with anti-CD3 and anti-CD28 under indicated conditions and treated with an endosome inhibitor, Latrunculin B (Lat B), for 48 h. (c) mRNA expression of Th2-specific genes was analysed by qRT–PCR. (d) IL-4R protein expression was analysed by FACS. Numbers in dot plot quadrants represent the percentages. The data shown ina,bandcwere normalized by the expression of a reference geneActb. The results shown are mean±s.e.m. *P<0.05, **P<0.01, Student’st-test was performed to detect between-group differences. The data are representative of at least three independent experiments with consistent results. Figure 4: Grail controls IL-4 receptor expression in Th2 cells. ( a ) Naïve CD4 + T cells from WT and Grail KO mice were activated with anti-CD3 and anti-CD28 in the presence or absence of IL-4 for 24, 48 and 72 h and analysed for expression of Il2 and Il21 by qRT–PCR. ( b ) Naïve CD4 + T cells from WT and Grail KO mice were activated with anti-CD3 and anti-CD28 along with the indicated conditions for 48 h and the mRNA expression of the indicated genes was analysed. ( c , d ) Naïve CD4 + T cells from WT mice were activated with anti-CD3 and anti-CD28 under indicated conditions and treated with an endosome inhibitor, Latrunculin B (Lat B), for 48 h. ( c ) mRNA expression of Th2-specific genes was analysed by qRT–PCR. ( d ) IL-4R protein expression was analysed by FACS. Numbers in dot plot quadrants represent the percentages. The data shown in a , b and c were normalized by the expression of a reference gene Actb . The results shown are mean±s.e.m. * P <0.05, ** P <0.01, Student’s t -test was performed to detect between-group differences. The data are representative of at least three independent experiments with consistent results. Full size image Grail controls Th2 responses in vivo To analyse the function of Grail in vivo, FACS-sorted memory CD4 + CD44 hi T cells from WT and Grail KO mice were analysed. As measured by quantitative reverse transcription–PCR (qRT–PCR), Grail-deficient CD4 + CD44 hi effector memory cells had significantly higher expression of major Th2-specific genes like Il4 and its receptor ( Supplementary Fig. 5a ) compared with WT cells. Higher IL-4, IL-5 and IL-13 protein levels were also detected by ELISA in the Grail-deficient memory cells compared with WT cells ( Supplementary Fig. 5b ), supporting Grail as an essential factor in Th2 differentiation in vivo. To further determine the role of Grail in Th2 responses in vivo , WT and Grail KO mice were immunized intraperitoneally with ovalbumin (Ova) and the adjuvant aluminium hydroxide (alum). After restimulation with Ova, T cells from Grail KO mice had significantly higher expression of IL-2, IL-4, IL-5 and IL-13 ( Fig. 5a ). Similarly, intracellular staining revealed a dramatic increase in CD4 + IL-4 + cells in both the spleen and lung lymph nodes of Grail KO mice compared with WT mice ( Fig. 5b ). In addition, analysis of sorted CD4 + CD44 hi cells from immunized mice showed that Grail deficiency led to enhanced expression of Th2-specific factors (IL-4, IL-5, IL-13 and Gata3) both at mRNA and protein levels ( Fig. 5c ). 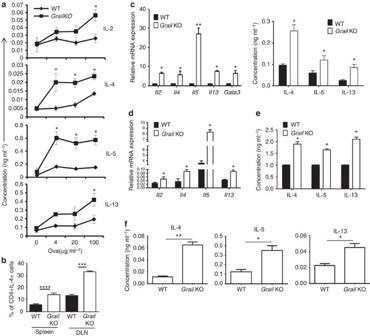Figure 5: Grail deficiency leads to saturated Th2 responsesin vivo. (a–c) Male WT andGrailKO mice (6–8 weeks,n=5 per group) were intraperitoneally injected with Ova in alum. (a) Seven days after immunization, splenocytes were restimulated with different concentrations of Ova and Th2 cytokines were measured by ELISA. (b) Percentage of Ova-specific CD4+IL-4+cells in spleen and lung lymph nodes of WT andGrailKO mice. (c) CD4+CD44hicells were sorted from the spleen and lung lymph nodes of immunized mice and expression of Th2 genes was analysed by qRT–PCR and ELISA. The data shown were normalized by the expression of a reference geneActb. (d,e) FACS sorted naïve CD4+T cells from WT andGrailKO mice were intravenously transferred intoTCR-β KO mice (5 million cells per mouse,n=4 per group) followed by intraperitoneal injection with Ova in alum. Seven days later WT andGrailKO CD4+CD44hicells were sorted and effector cytokine levels were measured by qRT–PCR analysis (d) and ELISA (e). (f) Mixed–bone marrow chimeric mice (n=10) were generated by co-transfer of 10 million cells at a ratio of 1:1 WT (CD45.2) andGrailKO (CD45.1) bone marrow cells intoRag1KO mice. Eight weeks later, mice were immunized with Ova in alum. One week later, WT andGrailKO CD4+CD44hicells were sorted and effector cytokine levels were measured by ELISA. The results shown are mean±s.e.m. *P<0.05, **P<0.01, ***P<0.001, ****P<0.0001, Student’st-test was performed to detect between-group differences. The data are representative of at least three independent experiments with consistent results. Figure 5: Grail deficiency leads to saturated Th2 responses in vivo . ( a – c ) Male WT and Grail KO mice (6–8 weeks, n =5 per group) were intraperitoneally injected with Ova in alum. ( a ) Seven days after immunization, splenocytes were restimulated with different concentrations of Ova and Th2 cytokines were measured by ELISA. ( b ) Percentage of Ova-specific CD4 + IL-4 + cells in spleen and lung lymph nodes of WT and Grail KO mice. ( c ) CD4 + CD44 hi cells were sorted from the spleen and lung lymph nodes of immunized mice and expression of Th2 genes was analysed by qRT–PCR and ELISA. The data shown were normalized by the expression of a reference gene Actb . ( d , e ) FACS sorted naïve CD4 + T cells from WT and Grail KO mice were intravenously transferred into TCR- β KO mice (5 million cells per mouse, n =4 per group) followed by intraperitoneal injection with Ova in alum. Seven days later WT and Grail KO CD4 + CD44 hi cells were sorted and effector cytokine levels were measured by qRT–PCR analysis ( d ) and ELISA ( e ). ( f ) Mixed–bone marrow chimeric mice ( n =10) were generated by co-transfer of 10 million cells at a ratio of 1:1 WT (CD45.2) and Grail KO (CD45.1) bone marrow cells into Rag1 KO mice. Eight weeks later, mice were immunized with Ova in alum. One week later, WT and Grail KO CD4 + CD44 hi cells were sorted and effector cytokine levels were measured by ELISA. The results shown are mean±s.e.m. * P <0.05, ** P <0.01, *** P <0.001, **** P <0.0001, Student’s t -test was performed to detect between-group differences. The data are representative of at least three independent experiments with consistent results. Full size image To check whether the increased Th2 responses in Grail KO mice are T-cell intrinsic, we transferred naïve WT and Grail KO CD4 + cells into TCR- β KO mice followed by Ova in alum immunization. Consistent with above data, mice reconstituted with Grail KO CD4 + T cells showed increased expression of Th2 cytokines both at mRNA and protein levels compared with mice that received WT CD4 + T cells ( Fig. 5d,e ). To further demonstrate the role of Grail in T cells, we generated mixed bone marrow chimeras by transferring a mixture of congenic CD45.1 + WT and CD45.2 + Grail-deficient bone marrow cells into sub-lethally irradiated Rag1 KO mice. Eight weeks after reconstitution, we immunized mice with Ova protein in alum. CD4 + CD44 hi Grail-deficient cells exhibited enhanced Th2-specific cytokine expression compared with WT cells ( Fig. 5f ). The above results confirm that Grail expression in T cells is required to control Th2 programming in vivo. As Th2 cells are pathogenic, we next subjected WT and Grail KO mice to allergic asthma using a standard protocol [21] . Histology analysis revealed that Grail deficiency resulted in significantly more inflammatory cell infiltration into the lung tissue ( Fig. 6a ). Consistent with histological analysis, the numbers of total cells, eosinophils, neutrophils and lymphocytes in bronchoalveolar lavage fluid (BALF) were significantly increased in Grail KO mice compared with WT mice ( Fig. 6b ). In addition, we also observed increased levels of Th2 cytokines in BALF and lungs of Grail KO mice compared with their WT counterparts ( Fig. 6c,d ). Moreover, after restimulation ex vivo with Ova protein, spleen- and lung-associated lymph node cells from Grail KO mice produced more Th2 cytokines than did cells from WT mice ( Fig. 6e–g and Supplementary Fig. 5c ), suggesting that Grail is required to control the generation of proallergic helper T cells. 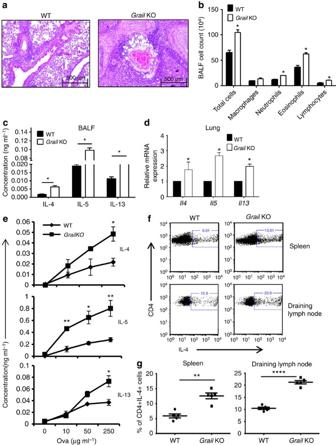Figure 6: Grail-deficient mice are more susceptible to allergic asthma. Groups of WT andGrailKO mice (6–8 weeks,n=5 per group) were intraperitoneally sensitized with Ova in alum with 2 weeks interval, followed by intranasal challenge with Ova. (a) Mononuclear cell infiltration in lung tissues from WT andGrailKO mice subjected to asthma was analysed by H&E staining. Original magnification × 20. Scale bar, 1 cm=500 μm. (b) Bronchoalveolar lavage fluids (BALFs) were analysed to measure airway infiltrating cells. (c) Protein levels of Th2 cytokines in BALF was analysed by ELISA. (d) mRNA expression of effector cytokines in the lungs of asthmatic WT andGrailKO mice were analysed by qRT–PCR. The data shown were normalized by the expression of a reference geneActb. (e) Lung lymph node cells from WT andGrailKO mice were restimulated with different concentrations of Ova and Th2 cytokines were measured by ELISA. (f) IL-4 expression by CD4+T cells from lung lymph nodes of WT andGrailKO mice following Ova restimulation was accessed by intracellular cytokine staining. Numbers in dot plot quadrants represent the percentages. (g) The percentage of CD4+IL-4+cells in the spleen and lung lymph nodes of asthmatic WT andGrailKO mice. The results shown inb–eare mean±s.e.m. *P<0.05, **P<0.01, Student’st-test was performed to detect between-group differences. The data are representative of at least three independent experiments with consistent results. Figure 6: Grail-deficient mice are more susceptible to allergic asthma. Groups of WT and Grail KO mice (6–8 weeks, n =5 per group) were intraperitoneally sensitized with Ova in alum with 2 weeks interval, followed by intranasal challenge with Ova. ( a ) Mononuclear cell infiltration in lung tissues from WT and Grail KO mice subjected to asthma was analysed by H&E staining. Original magnification × 20. Scale bar, 1 cm=500 μm. ( b ) Bronchoalveolar lavage fluids (BALFs) were analysed to measure airway infiltrating cells. ( c ) Protein levels of Th2 cytokines in BALF was analysed by ELISA. ( d ) mRNA expression of effector cytokines in the lungs of asthmatic WT and Grail KO mice were analysed by qRT–PCR. The data shown were normalized by the expression of a reference gene Actb . ( e ) Lung lymph node cells from WT and Grail KO mice were restimulated with different concentrations of Ova and Th2 cytokines were measured by ELISA. ( f ) IL-4 expression by CD4 + T cells from lung lymph nodes of WT and Grail KO mice following Ova restimulation was accessed by intracellular cytokine staining. Numbers in dot plot quadrants represent the percentages. ( g ) The percentage of CD4 + IL-4 + cells in the spleen and lung lymph nodes of asthmatic WT and Grail KO mice. The results shown in b – e are mean±s.e.m. * P <0.05, ** P <0.01, Student’s t -test was performed to detect between-group differences. The data are representative of at least three independent experiments with consistent results. Full size image Grail controls Stat6 expression in Th2 cells The above results suggest that Grail deficiency leads to Th2-hyperresponsiveness and Th2-mediated inflammation. Recently, we reported that Grail regulates CD4 + T-cell activation by targeting TCR-CD3 complex via proteasome-mediated degradation [21] . Owing to its high expression in Th2 cells, first we assessed whether Grail controls Th2 cells by targeting CD3ζ. However, analysis of TCRβ downregulation in WT and Grail KO Th2 cells upon anti-CD3 stimulation did not show difference in TCRβ levels between WT and Grail KO cells ( Supplementary Fig. 6 ). Next, we analysed the protein level of Th2 transcriptional factors such as Stat6 and Gata3 in naïve WT and Grail KO CD4 + T cells either left unstimulated or stimulated with anti-CD3/28 in the presence or absence of IL-4 ( Fig. 7a and Supplementary Fig. 10a ). Stat6 protein levels were increased in naïve CD4 + T cells in Grail KO mice compared with WT mice. This increase was maintained after 24 h of anti-CD3/28 stimulation either in the presence or absence of IL-4 ( Fig. 7a and Supplementary Fig. 10a ). Moreover, fully committed Th2 cells from Grail KO mice showed a more dramatic increase in Stat6 protein expression ( Fig. 7b and Supplementary Fig. 10b ). In addition to Stat6, Gata3 protein expression was also significantly enhanced in Grail-deficient Th2 cells ( Fig. 7b and Supplementary Fig. 10b ), whereas we did not detect enhanced Gata3 protein level at early steps of Th2 development ( Supplementary Figs 9 and 10g ), suggesting that Grail potentially controls Gata3 expression through Stat6. To further dissect the expression and activation kinetics of Stat6 in IL-4-primed cells, we isolated naïve CD4 + T cells from WT and Grail KO mice and activated them with anti-CD3/28 and IL-4 for different time points. Interestingly, analysis of phospho-Stat6 level revealed significant activation of Stat6 in Grail-deficient T cells activated in the presence of only anti-CD3/28 compared with WT cells ( Fig. 7c and Supplementary Fig. 10c ). This increase was further enhanced in the presence of IL-4. The total Stat6 levels were also increased in Grail-deficient T cells ( Fig. 7c and Supplementary Fig. 10c ), suggesting that Grail may regulate Th2 programming by targeting Stat6. 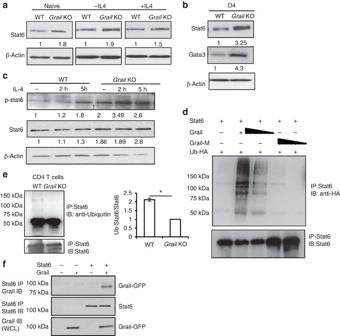Figure 7: Grail negatively regulates Stat6 expression and activity. (a) Naïve CD4+T cells from WT andGrailKO mice were activated with anti-CD3/anti-CD28 in the presence or absence of IL-4 for 24 h, and Stat6 protein expression were detected by western blot analysis. (b) Naive CD4+T cells from WT andGrailKO mice were cultured for 4 days under Th2 differentiation conditions and analysed for Stat6 and Gata3 expression by western blot analysis. The numbers inaandbdepict relative immune blotting signals compared with WT after normalizing with β-actin levels. (c) Naive CD4+T cells from WT andGrailKO mice were isolated and serum starved for 12 h followed by activation with anti-CD3/ant-CD28 in the presence or absence of IL-4 for the indicated time points and phospho-Stat6 and total Stat6 levels were determined by western blot analysis. β-Actin levels were determined in the same samples as loading control. The numbers depict relative immune blotting signals compared with WT anti-CD3/CD28 only treated samples after normalizing with β-actin levels. (d) HEK293T cells were transfected with vectors encoding Stat6, HA-Ub and either Grail or a Grail mutant. The lysates were subjected to immunoprecipitation (IP) using anti-Stat6 antibody. The blot was probed with anti-HA-HRP and re-probed for Stat6 expression. (e) CD4+T cells from WT andGrailKO mice were activated with anti-CD3 and IL-4 along with MG132 (proteasome inhibitor) for 6 h. The cell lysates were then immunoprecipitated using anti-Stat6 antibody and the blot was probed with anti-ubiquitin or anti-Stat6 antibodies. Relative western blotting signals were calculated as a ratio of ubiquitinated and non-ubiquitinated Stat6. (f) HEK293T cells were either left untransfected or transfected with vectors encoding Stat6, Grail-GFP or both. The lysates were subjected to IP using anti-Stat6 antibody. The blot was probed with anti-GFP antibody (upper panel) and re-probed with anti-Stat6 antibody (middle panel) as a control. The WCL was immunoblotted with anti-GFP antibody (lower panel) for checking antibody efficacy. The results shown in the figures are representative blots of at least three independent experiments. *P<0.05, Student’st-test was performed to detect between-group differences. Figure 7: Grail negatively regulates Stat6 expression and activity. ( a ) Naïve CD4 + T cells from WT and Grail KO mice were activated with anti-CD3/anti-CD28 in the presence or absence of IL-4 for 24 h, and Stat6 protein expression were detected by western blot analysis. ( b ) Naive CD4 + T cells from WT and Grail KO mice were cultured for 4 days under Th2 differentiation conditions and analysed for Stat6 and Gata3 expression by western blot analysis. The numbers in a and b depict relative immune blotting signals compared with WT after normalizing with β-actin levels. ( c ) Naive CD4 + T cells from WT and Grail KO mice were isolated and serum starved for 12 h followed by activation with anti-CD3/ant-CD28 in the presence or absence of IL-4 for the indicated time points and phospho-Stat6 and total Stat6 levels were determined by western blot analysis. β-Actin levels were determined in the same samples as loading control. The numbers depict relative immune blotting signals compared with WT anti-CD3/CD28 only treated samples after normalizing with β-actin levels. ( d ) HEK293T cells were transfected with vectors encoding Stat6, HA-Ub and either Grail or a Grail mutant. The lysates were subjected to immunoprecipitation (IP) using anti-Stat6 antibody. The blot was probed with anti-HA-HRP and re-probed for Stat6 expression. ( e ) CD4 + T cells from WT and Grail KO mice were activated with anti-CD3 and IL-4 along with MG132 (proteasome inhibitor) for 6 h. The cell lysates were then immunoprecipitated using anti-Stat6 antibody and the blot was probed with anti-ubiquitin or anti-Stat6 antibodies. Relative western blotting signals were calculated as a ratio of ubiquitinated and non-ubiquitinated Stat6. ( f ) HEK293T cells were either left untransfected or transfected with vectors encoding Stat6, Grail-GFP or both. The lysates were subjected to IP using anti-Stat6 antibody. The blot was probed with anti-GFP antibody (upper panel) and re-probed with anti-Stat6 antibody (middle panel) as a control. The WCL was immunoblotted with anti-GFP antibody (lower panel) for checking antibody efficacy. The results shown in the figures are representative blots of at least three independent experiments. * P <0.05, Student’s t -test was performed to detect between-group differences. Full size image To check whether Grail directly targets Stat6, we overexpressed Stat6 together with WT or Grail mutant, which lacks amino acids encompassing the RING domain (amino acids 277–317) and hence the E3 ubiquitin ligase activity in HEK293T cells along with HA-tagged ubiquitin. After immunoprecipitation of Stat6 with Stat6 antibody and re-probing with HA-HRP antibodies, we observed the formation of higher molecular weight ubiquitin conjugates in the presence of WT Grail, indicating polyubiquitin chain formation ( Fig. 7d and Supplementary Fig. 10d ). This ubiquitination was decreased upon lowering the concentration of WT Grail and was not present upon overexpression of the Grail mutant ( Fig. 7d and Supplementary Fig. 10d ). Thus, Stat6 is a potential substrate for Grail-mediated ubiquitination in Th2 cells. In further investigation, we checked the endogenous ubiquitination of Stat6 in WT and Grail-deficient CD4 + T cells activated with anti-CD3/28 and IL-4 in the presence of MG132 to block any proteasome degradation. T-cell lysates were then immunoprecipitated with Stat6 antibodies and immunoblotted with ubiquitin antibodies. Compared with WT cells, ubiquitination of Stat6 in Grail-deficient cells was substantially reduced ( Fig. 7e and Supplementary Fig. 10e ), suggesting that Grail regulates Stat6 expression and function through ubiquitin-dependent proteasome degradation pathway. Moreover, immunoprecipitation experiments performed in HEK293T cells transfected with expression vectors for Stat6 and Grail-GFP revealed an interaction between Grail and Stat6 ( Fig. 7f and Supplementary Fig. 10f ), thus suggesting that ubiquitination of Stat6 by Grail is mediated by their physical interaction. However, we were unable to detect interaction between endogenous Grail and Stat6 proteins because of unavailability of efficient Grail antibodies. Further experiments with the endogenous Grail would be required to establish the physical interaction between Grail and Stat6 in a physiological setting. The molecular mechanisms leading to generation of pro-allergenic Th2 cells are gradually becoming clearer. Although most of the previous studies have focused on active regulators of the Th2 differentiation programme, including transcription factors like Stat6, Gata3, JunB, IRF4, c-Maf and NFAT [7] , the mechanisms that keep Th2 cell generation and function under control remain poorly understood. In the current study, we have shown the essential role of Grail in regulating Th2 cell development and Th2-mediated pathogenic responses. Grail is preferentially expressed in Th2 cells, targets Stat6 for ubiquitination and restricts expression of Th2 cytokines. As a result, Grail-deficient mice are more susceptible to Th2-dependent allergic responses like asthma. It has been reported that Grail mRNA is upregulated during normal T-cell activation even under non-tolerant conditions [21] , [22] . As reported previously [23] , our analysis of Grail expression in in vitro differentiated different Th subsets showed that Grail is highly expressed in Th2 cells, suggesting the potential role of Th2 cytokines in regulation of Grail expression ( Fig. 1a ). We tested a panel of cytokines that are known to promote Th2 development including IL-2, IL-4 and IL-21 (refs 1 , 17 , 18 , 26 ) and found that Grail expression selectively depends on the presence of IL-4 ( Supplementary Fig. 8a ). Consistent with that, upon IL-4 blockade, T cells stimulated with ant-CD3 and CD28 failed to upregulate Grail expression ( Fig. 1c ). Moreover, we observed correlation between Grail and Il4 expression ( Fig. 1c and Supplementary Fig. 7 ), which suggests that Grail could serve as a marker of pro-allergic cells where IL-4 signalling determines Grail expression. In fact, Stat6 and Gata3, major Th2-specific transcription factors [7] , bind to and transactivate the Grail promoter ( Fig. 2e ) and are necessary and sufficient to induce Grail as evident from overexpression experiments ( Fig. 2d ). Higher Grail expression was also detected in Th9 cells ( Supplementary Fig. 8b ). This could be mediated by the IL-4-IL-4R-Stat6 signalling pathway, which is important for the development of Th9 cells as well [27] , [28] . In addition to Stat6 and Gata3, transcription factors like JunB and IRF4 are also known to be involved in the Th2 developmental process; however, they did not contribute to Th2-specific Grail expression ( Fig. 2c,d ). Previously, it has been proposed that NFATc1 has the potential to induce Grail in anergic T cells [29] . However, blockade of NFATc1 activity by CsA during Th2 development did not affect Grail expression and we did not detect transactivation of Grail promoter activity by overexpression of NFATc1 ( Supplementary Fig. 2d,e ). It is also possible that NFATc1 could cooperate with Stat6 and Gata3 to enhance and stabilize Grail expression in Th2 cells. As Grail is induced in Th2 cells by IL-4 signalling, Grail may be involved in the differentiation of Th2 cells. Indeed, Grail-deficiency in CD4 + T cells enhanced Th2-biased differentiation in vitro and in vivo ( Figs 3 , 5 and 6 ). Interestingly Il4r expression was also enhanced in the Grail-deficient T cells 24 h after IL-4 treatment and peaked at 48 h, suggesting the role of Grail in early stages of Th2 cell programming by regulating Il4r expression ( Fig. 3d,e and Supplementary Fig. 4a ). Moreover, analysis of naïve CD4 + T cells from Grail-deficient mice revealed that the Il4r promoter region is enriched in both permissive H3K4me3 and the restrictive H3K27me3 modifications ( Supplementary Fig. 3 ). This bivalent chromatin could allow minimal IL-4R expression in naïve cells but nonetheless make it poised for rapid transcriptional activation in response to subsequent IL-4 signalling favouring Th2 differentiation. IL-2 and IL-21 are known to aid in early events of Th2 cell differentiation [17] . We found that Grail-deficient CD4 + T cells expressed substantially high amounts of IL-2 and IL-21 compared with WT cells 24 h after IL-4 treatment ( Fig. 4a ). In addition, these cytokines facilitate the rapid expression of Il4r and Th2 cytokines in Grail-deficient CD4 + T cells. Our studies for the first time indicate a critical role of Grail in controlling of Il4r expression and Th2 programming. Our previous studies as well as others indicate that Grail negatively regulates T-cell responses by targeting components of TCR signalling pathway for degradation [21] , [22] . However, analysis of TCRβ downregulation in WT and Grail-deficient Th2 cells upon anti-CD3 stimulation did not show difference in TCRβ levels between WT and Grail KO cells ( Supplementary Fig. 6 ), indicating that TCR signalling is not responsible for the profound Th2 phenotype in Grail-deficient cells. Next, we analysed the protein level of Th2 transcriptional factors such as Stat6 and Gata3 in naïve and IL-4-treated WT and Grail KO CD4 + T cells. We found increased Stat6 protein level in naïve Grail KO CD4 + T cells compared with WT cells and this increase was maintained in Grail KO cells upon IL-4 stimulation ( Fig. 7a,b and Supplementary Fig. 10a,b ). We further determined that Grail interacts with Stat6 ( Fig. 7f and Supplementary Fig. 10f ) and the downregulation of elevated Stat6 levels by Grail is dependent on E3 ligase activity and mediated by proteasome-mediated degradation ( Fig. 7d,e and Supplementary Fig. 10d-e ). This result suggests that Grail, located in endosomal compartment, may target Stat6 via ubiquitination and proteasome-mediated degradation. Increased level of Stat6 could explain why Grail-deficient cells can spontaneously acquire a Th2 phenotype. In fact, we saw significantly enhanced Gata3 expression in fully polarized Grail-deficient Th2 cells compared with WT cells ( Fig. 7b and Supplementary Fig. 10b ). The augmented total Stat6, phospho-Stat6 and Gata3 levels in the absence of Grail could further lead to increase in the transcription of Th2 signature cytokines by direct binding to their promoters or by regulating the chromatin accessibility to other trans-activating factors. We also found increased abundance of active histone markers (AcH3 and H3k4) and decreased levels of suppressive markers (H3k27) in the Il4 , Il4r and Gata3 promoter locus in Grail KO Th2 cells ( Supplementary Fig. 3 ). Stat6 is known to influence the expression of an array of genes by regulating their chromatin structure [30] . Further investigation is needed to check whether Grail directly targets and influences the expression and functional status of chromatin modifiers involved in Th2 gene expression. In summary, our studies for the first time indicate the Th2-specific expression of Grail and its critical role in controlling Th2 responses. Grail expression is mainly mediated by IL-4 and IL-4 signalling components. It controls Th2 responses by targeting Stat6 transcription factor for degradation in activated Th2 cells. Thus, the results suggest Grail as a potential marker of allergic inflammation and provide a molecular mechanism explaining the generation of peripheral Th2 tolerance, which has implications in the prevention and treatment of allergic diseases. In addition to Grail, other E3 ubiquitin ligases such as Itch has been implicated in regulation of Th2 development by targeting JunB [31] . These E3 ligases could potentially cooperate with each other to play a synergistic role in promoting Th2 cell tolerance. Future studies in mice deficient in both Grail and Itch will potentially have therapeutic implications for allergic diseases. Mice and cell lines Grail KO mice were generated as described before [21] . OT II TCR transgenic, TCR-β KO, Rag1 KO, Stat6 KO and C57BL/6J mice were obtained from Jackson laboratory. All mice were housed in the SPF animal facility at M.D. Anderson Cancer Center and the animal experiments were performed using protocols approved by Institutional Animal Care and Use Committee. The EL4 (murine lymphoma) and HEK293T (human fibroblast) cell lines were purchased from ATCC and maintained in DMEM medium supplemented with 10% fetal bovine serum and antibiotics. T-cell differentiation T-cell differentiation was performed as described previously [21] , [32] . In brief, naïve CD4 + CD25 - CD62L hi CD44 lo T cells were flow cytometry-sorted from lymph nodes and spleens of various mice and activated with anti-CD3 and anti-CD28 (BD Pharmingen, 2 μg ml −1 ) under Th0 (hIL-2-Peprotech, 50 U ml −1 ), Th1 (anti-IL-4-Bioexcel,10 μg ml −1 , IL-12-Peprotech, 10 ng ml −1 , hIL-2-50 U ml −1 ), Th2 (anti-IFN-γ-Bioexcel,10 μg ml −1 , IL-4-Peprotech, 10 ng ml −1 , hIL-2-50 U ml −1 ) and Th17 (anti-IFN-γ-10 μg ml −1 , anti-IL-4-10 μg ml −1 , IL-6-Peprotech, 20 ng ml −1 , TGF-β-Peprotech, 20 ng ml −1 ) polarizing conditions for 4 days. Cells were restimulated with anti-CD3 for 4 h before mRNA analysis qRT–PCR Total RNA was prepared from naïve or differentiated T cells using TriZol reagent (Invitrogen). cDNA was synthesized using Superscript reverse transcriptase and oligo(dT) primers (Invitrogen), and gene expression of β-actin ( Actb ), Grail , Il21 , Il4 , Gata3 (refs 21 , 33 , 34 ), Il2 (F: 5′-GCGCACCCACTTCAAGCTCCA-3′; R: 5′-CTGTGGCCTGCTTGGGCAAGT-3′), Il5 (F: 5′-CGCTCACCGAGCTCTGTTG-3′; R: 5′-CCAATGCATAGCTGGTGATTTTT-3′), Il13 (F: 5′-GCTTATTGAGGAGCTGAGCAACA-3′; R: 5′-GGCCAGGTCCACACTCCATA-3′) and Stat6 (F: 5′-AGTCACTATAAGCCCGAACAG-3′; R: 5′-GCCATTCCAAGATCATAAGGT-3′) was examined with a Bio-Rad iCycler Optical System using iQ SYBR green real-time PCR kit (Bio-Rad Laboratories, Inc.). The data were normalized to β-Actin gene. Retroviral transduction Retroviral transduction was performed as described previously [21] . Briefly, naive CD4 + CD25 - CD62L hi CD44 lo T cells from OT-II mice were sorted by flow cytometry and activated with Ova peptide and irradiated WT splenic antigen-presenting cells. Twenty-four hours after activation, cells were infected by retroviruses expressing Stat6, Gata3, IRF4 or JunB or control empty vector (containing only IRES-GFP). Four days after infection, GFP + cells were flow cytometry-sorted and restimulated with anti-CD3 for 4 h, and mRNA expression levels were analysed by qRT–PCR analysis. For overexpression experiments in Fig. 2f and Supplementary Fig. 2b, naive CD4 + CD25 - CD62L hi CD44 lo T cells were sorted by flow cytometry from C57BL/6J (WT) and Stat6 KO mice by flow cytometry and activated with anti-CD3 and anti-CD28 for 24 h before infection. ChIP assay Naive CD4 + CD25 - CD62L hi CD44 lo T cells were isolated and activated under Th0 or Th2 differentiation conditions. Four days later cells were restimulated with anti-CD3 (2 μg ml −1 ) for 4 h and fixed with 1% formaldehyde for 10 min at 37 °C. ChIP was performed using the Millipore ChIP kit. Briefly, chromatin was seared (500 bp–100 kb) and immunoprecipitated using the antibodies to the following: AcH3 (06–599), H3k4me3 (07–473), H3k27me3 (074–449), Rabbit IgG (12–370) (Millipore, 2.5 μg per sample), Stat6 (sc-981), IRF4 (sc-6059), JunB (sc-73) and Gata3 (sc-22206) (Santa Cruz Biotechnology, 5 μg per sample). Following reversal of cross-links, the presence of selected DNA sequences was assessed by qRT–PCR using the following primer sequences: Grail promoter (primer1—F: 5′-TTTTAAGAGGCGGATCCCGCA-3′; R: 5′-GCTGGGACTAGGTGCGAACCAG-3′); primer 2—F: 5′-AAATCGAGGCGCAGAGAAGTAA-3′; R: 5′-CTAAAATGAGGCCAGCCCACCT-3′), Il4 promoter (Histone and Stat6 ChIP, respectively) [35] , [36] , HS2 locus [37] , CNS-3 (IL-10 locus) [38] , CNS+6.45 (IL-10 locus) [39] . Immunoblot (IB) analysis and ubiquitination assay Western blot analysis and ubiquitination assay were performed as described previously [21] . Briefly, whole T-cell lysates were prepared by lysing cells in triton lysis buffer. The amounts of protein were determined by Bio-Rad protein assay (Bio-Rad) to ensure equal protein loading for IB analysis with antibodies to Stat6, phospho-Stat6 and Gata3 (Santa Cruz Biotechnology, 1:1,000 dilution) and β-Actin (Pierce, 1:1,000 dilution). For ubiquitination assays, HEK293T cells were transfected in six-well plates with retroviral expression vector containing Stat6 (kindly provided by Mark Boothby, Vanderbilt University); bicistronic retroviral vector pGFP-RV containing either Grail or Grail mutant (Grail-M) and pcDNA-HA-ubiquitin. Stat6 protein in the cell lysates was immunoprecipitated using anti-Stat6 antibody (5 μg per sample), followed by detection of ubiquitinated Stat6 by IB using anti-HA-HRP (Santa Cruz Biotechnology, 1:1,000 dilution). For detecting endogenous ubiquitination of Stat6, cells were lysed in kinase lysis buffer supplemented with 1 mM N -ethylmaleimide. Stat6 protein was immunoprecipitated using Stat6-specific antibody, and the ubiquitin-conjugated Stat6 was detected by IB using anti-ubiquitin (Santa Cruz Biotechnology, 1:500 dilution). For co-immunoprecipitation experiments, HEK293T cells were transfected in six-well plates with retroviral expression vectors containing Stat6 and Grail-GFP. Stat6 protein in the cell lysates was immunoprecipitated using anti-Stat6 antibody (5 μg per sample), followed by detection of Grail by IB using anti-GFP antibody (Santa Cruz Biotechnology, 1:500 dilution). Ova immunization Male WT (C57BL/6J) and Grail KO mice (6–8 weeks old, n =5 per group) were immunized with Ova protein (1.0 mg ml −1 ) emulsified in alum intraperitoneally. Seven days after immunization, mice were killed and analysed individually. Spleen cells from Ova-immunized mice were stimulated in 96-well plates as triplicates with or without different concentrations of Ova protein. IL-2 production was determined 24 h after T-cell activation by ELISA. Effector cytokines were analysed 3 days later by ELISA (PharMingen). Adoptive transfer and mixed bone marrow chimera studies Adoptive transfer and bone marrow chimera experiments were done as described previously [40] . Briefly, FACS-sorted naïve CD4 + T cells from 8-week-old male WT or Grail KO mice were intravenously transferred into 6- to 8-week-old male TCR- β KO mice (10 × 10 6 cells per mouse, n =4 per group). The recipient mice were immunized i.p. with Ova in alum 24 h post transfer. Seven days after immunization, spleen cells from the recipient mice were isolated and CD4 + CD44 hi effector memory cells were sorted for analysis. To generate mixed bone marrow chimera, T-cell-depleted bone marrow cells were obtained from 6- to 8-week-old male B6.SJL (CD45.1) or Grail KO mice and mixed 1:1 ratio before being transferred into irradiated male (6–8 weeks old, n =10) Rag1 KO mice (10 × 10 6 cells per mouse, 750 rad). Eight weeks later, the recipient mice were immunized with Ova in alum and analysed as above. Asthma induction Asthma induction was done as described previously [21] , [41] . Breifly, male WT (C57BL/6J) and Grail KO mice (6–8 weeks old, n =5per group) were immunized twice intraperitoneally at 2 weeks interval with 0.2 ml saline containing 100 μg Ova in alum. On day 14, mice were intranasally challenged with Ova followed by three more challenges on days 26, 27 and 28. After 24 h, the last challenge mice were killed and the BALF, lungs, spleens and the lung lymph nodes were harvested for further analysis. Statistical analysis The results shown are mean±s.e.m. Student’s t -test was performed to detect between-group differences. A P value of <0.05 was rendered statistically significant. * P <0.05, ** P <0.01, *** P <0.001 and **** P <0.0001. How to cite this article: Sahoo, A. et al. Grail controls Th2 cell development by targeting STAT6 for degradation. Nat. Commun. 5:4732 doi: 10.1038/ncomms5732 (2014).